Assessing technical performance in differential gene expression experiments with external spike-in RNA control ratio mixtures There is a critical need for standard approaches to assess, report and compare the technical performance of genome-scale differential gene expression experiments. Here we assess technical performance with a proposed standard ‘dashboard’ of metrics derived from analysis of external spike-in RNA control ratio mixtures. These control ratio mixtures with defined abundance ratios enable assessment of diagnostic performance of differentially expressed transcript lists, limit of detection of ratio (LODR) estimates and expression ratio variability and measurement bias. The performance metrics suite is applicable to analysis of a typical experiment, and here we also apply these metrics to evaluate technical performance among laboratories. An interlaboratory study using identical samples shared among 12 laboratories with three different measurement processes demonstrates generally consistent diagnostic power across 11 laboratories. Ratio measurement variability and bias are also comparable among laboratories for the same measurement process. We observe different biases for measurement processes using different mRNA-enrichment protocols. Ratios of mRNA transcript abundance between sample types are measures of biological activity. These measurements of differential gene expression are important to underpin new biological hypotheses and to support critical applications such as selection of disease classifiers and regulatory oversight of drug therapies. Controls and associated ratio performance metrics are essential to understand the reproducibility and validity of differential expression experimental results. External spike-in control ratio measurements can serve as a truth set to benchmark the accuracy of endogenous transcript ratio measurements. A library of 96 external RNA spike-in controls developed by the External RNA Controls Consortium (ERCC) [1] and distributed by NIST as Standard Reference Material 2374 (ref. 2 ) can act as technology-independent controls for differential expression experiments. Method validation of differential expression experiments based on these ERCC controls is the focus of this work. This validation supports comparisons across experiments, laboratories, technology platforms and data analysis methods [3] , [4] , [5] , [6] , [7] . In any differential expression experiment, with any technology platform, a pair of ERCC control ratio mixtures can be added (‘spiked’) into total RNA samples such that for each ERCC control the relative abundance of the control between samples (ratio) is either of known difference (a true-positive control) or the same (a true-negative control). To enable rapid, reproducible and automated analysis of any differential expression experiment we present a new software tool, the erccdashboard R package, which produces ERCC ratio performance metrics from expression values (for example, sequence counts or microarray signal intensities). These ratio performance measures include diagnostic performance of differential expression detection with receiver operating characteristic (ROC) curves and area under the curve (AUC) statistics, limit of detection of ratio (LODR) estimates and expression ratio technical variability and bias. Ratio performance measures provided by the erccdashboard package do not supersede other quality control (QC) measures, such as the QC methods recommended to evaluate sequence data both before and after alignment to a reference sequence in RNA-Seq experiments [8] , [9] , [10] , [11] , [12] . Sequence-level QC methods are important for evaluating the quality of data in both transcript-discovery and differential expression RNA-Seq experiments but do not provide the additional analysis of positive and negative controls to fully evaluate differential expression experiment technical performance. Analysis of ERCC ratio mixtures with the erccdashboard package provides technology-independent ratio performance metrics (applicable to RNA-Seq, microarrays or any future gene expression measurement technologies). These metrics are a significant extension beyond previous work with ERCC transcripts in RNA-Seq measurements [13] . In this earlier work, a single mixture of ERCC transcripts was used to assess dynamic range and precision in individual transcript-discovery RNA-Seq measurements. This earlier work did not assess differential expression experiments using ratio performance metrics from ERCC control ratio mixtures. The source to create ERCC ratio mixtures is a plasmid DNA library of ERCC sequences that is available as a standard reference material from NIST (SRM 2374 (ref. 2 )). This library of 96 sequences is intended for use as controls in commercial products, such as the pair of ERCC ratio mixtures used in this analysis. In these commercially available mixtures (Mix 1 and Mix 2), 92 of the 96 ERCC RNA molecule species were pooled to create mixes with true-positive and true-negative relative abundance differences. The two ERCC ratio mixtures are each composed of four subpools (23 ERCC controls per subpool) with defined abundance ratios between the mixes ( Fig. 1a ). Three of the subpools have different ERCC abundances in Mix 1 and Mix 2 (4:1, 1:2 and 1:1.5 ratios), and one subpool has identical ERCC abundances in the two mixes (a 1:1 ratio). Within each subpool ERCC abundances span a 2 20 dynamic range. 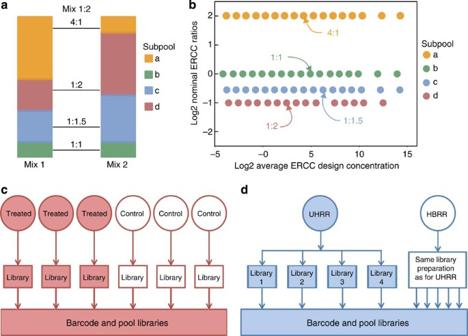Figure 1: Design of ERCC RNA control ratio mixtures and example experiments. (a) Two mixtures of the same 92 ERCC RNA transcripts are prepared such that four subpools with 23 transcripts per subpool are in four defined abundance ratios between the two mixtures. (b) Within each subpool the 23 controls (several points overlap) span a broad dynamic range of transcript concentrations. (c) In a typical single laboratory RNA-Seq experiment, biological replicates would be prepared for treatment and control samples. Rat toxicogenomics experimental samples represent this experimental design. (d) In the interlaboratory study design UHRR and HBRR samples have no biological replicates but have extensive technical replicates including multiple library preparation replicates that are analysed for the interlaboratory assessment of reproducibility instead of biological replicates. Figure 1b illustrates the ratio-abundance relationship of the 92 controls in the pair of mixtures. Figure 1: Design of ERCC RNA control ratio mixtures and example experiments. ( a ) Two mixtures of the same 92 ERCC RNA transcripts are prepared such that four subpools with 23 transcripts per subpool are in four defined abundance ratios between the two mixtures. ( b ) Within each subpool the 23 controls (several points overlap) span a broad dynamic range of transcript concentrations. ( c ) In a typical single laboratory RNA-Seq experiment, biological replicates would be prepared for treatment and control samples. Rat toxicogenomics experimental samples represent this experimental design. ( d ) In the interlaboratory study design UHRR and HBRR samples have no biological replicates but have extensive technical replicates including multiple library preparation replicates that are analysed for the interlaboratory assessment of reproducibility instead of biological replicates. Full size image Ratio mixture analysis with the erccdashboard is demonstrated for two types of differential expression studies: (1) rat toxicogenomics experiments with different treatments conducted at a single sequencing laboratory [14] and (2) interlaboratory analysis of the samples used in the MicroArray Quality-Control (MAQC) study [15] , Universal Human Reference RNA [16] (UHRR) and Human Brain Reference RNA (HBRR). The rat toxicogenomics study design consists of biological replicates for treatment and control conditions and illustrates a canonical RNA-Seq differential expression experiment with biological sample replication ( Fig. 1c ). In the interlaboratory study of the reference RNA samples, library replicates are compared in lieu of biological replicates ( Fig. 1d ). The interlaboratory study design offers a valuable opportunity to evaluate performance of experiments at individual laboratories and reproducibility between laboratories, even in the absence of biological replication because of the use of reference samples. Aliquots from a pair of spiked reference RNA samples were distributed to multiple laboratories for the Sequencing Quality-Control (SEQC) project [17] and the Association of Biomolecular Resource Facilities (ABRF) interlaboratory study [18] . Both studies measured the same samples on multiple measurement platforms. Subsets of experiments from these studies are analysed here with the erccdashboard package. These experiments include RNA-Seq experiments from the SEQC study using the Illumina HiSeq platform (ILM SEQC Lab 1–6) and the Life Technologies 5500 platform (LIF SEQC Lab 7–9), and ABRF study Illumina HiSeq platform (ILM ABRF Lab 10–12). Three laboratories in the SEQC project also performed microarray experiments with these same samples (Illumina BeadArray experiments at Lab 13 and 14 and a custom Agilent 1 M array at Lab 15). Analysis of a differential gene expression experiment using the erccdashboard package produces four main analysis figures. These four erccdashboard figures enable ‘reproducible research’ by providing an assessment of the key technical performance measures for any differential expression experiment. Examples of these four figures are presented for rat toxicogenomics experiments and reference RNA experiments from the large SEQC and ABRF experiment cohorts. Here we also evaluate the reproducibility of reference RNA experiments among laboratories using the SEQC and ABRF interlaboratory study data. Analysis of the sequencing experiments from the 12 laboratories participating in the interlaboratory study shows generally consistent diagnostic power across 11 out of the 12 participating laboratories. Ratio measurement variability and bias are also comparable among laboratories that used the same measurement process, which is defined here as a combination of sample preparation and sequencing. Three distinct measurement processes are assessed in this interlaboratory analysis and we observe different biases for measurement processes that include different mRNA-enrichment protocols. Examples of the erccdashboard performance measure figures are presented in Figs 2 , 3 , 4 , 5 for two arbitrarily-selected example experiments from the large SEQC and ABRF experiment cohorts (for all results see Supplementary Figs 1–20 ). These two examples are a rat toxicogenomics methimazole-treated (MET) and control (CTL) sample RNA-Seq experiment with biological replication ( Figs 2a–5a and Supplementary Fig. 2 ) and the Lab 5 RNA-Seq reference sample experiment ( Figs 2b–5b and Supplementary Fig. 10 ). 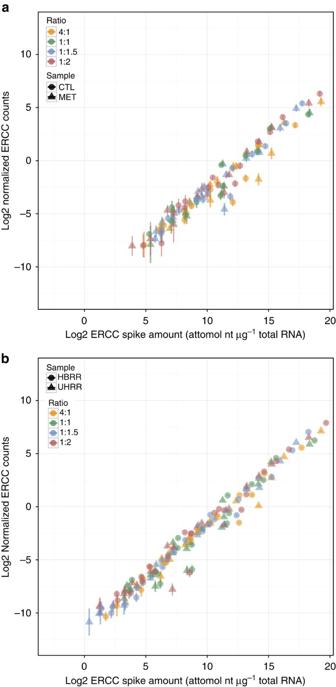Figure 2: Signal-abundance plots show dynamic range of experiments. (a) dynamic range of a rat toxicogenomics experiment with biological replicates (n=3) of control (CTL) and methimazole-treated (MET) (b) dynamic range of an RNA-Seq measurement of reference samples (UHRR and HBRR) with library preparation technical replicates (n=4) from Lab 5 of an interlaboratory study. In each figure points are coloured by ratio subpool, error bars represent the standard deviations of replicates, and shape represents sample type. In the RNA-Seq results, ERCC controls that did not have at least one count in three libraries for either sample were not included in the signal-abundance plot. Figure 2: Signal-abundance plots show dynamic range of experiments. ( a ) dynamic range of a rat toxicogenomics experiment with biological replicates ( n =3) of control (CTL) and methimazole-treated (MET) ( b ) dynamic range of an RNA-Seq measurement of reference samples (UHRR and HBRR) with library preparation technical replicates ( n =4) from Lab 5 of an interlaboratory study. In each figure points are coloured by ratio subpool, error bars represent the standard deviations of replicates, and shape represents sample type. In the RNA-Seq results, ERCC controls that did not have at least one count in three libraries for either sample were not included in the signal-abundance plot. 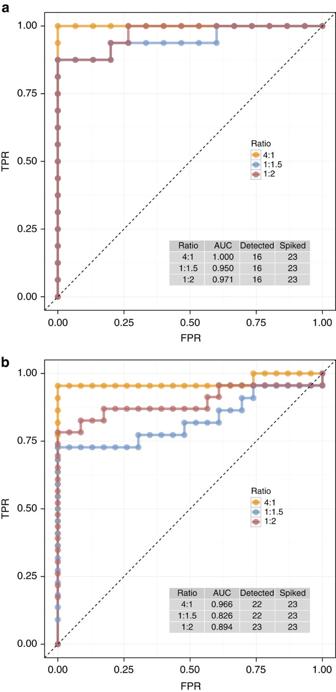Figure 3: ROC curves and AUC statistics show diagnostic performance of experiments. (a) Shown for biological replicates (n=3) of control (CTL) and methimazole-treated (MET) from a rat toxicogenomics experiment, (b) shown for an RNA-Seq measurement of reference samples (UHRR and HBRR) with library preparation technical replicates (n=4) from Lab 5 of an interlaboratory study. Annotation tables include AUC statistics for each group of true-positive ERCC controls along with the number of controls that were used in this analysis (‘detected’) and the total number that were included in the ERCC control mixtures (‘spiked’). Full size image Figure 3: ROC curves and AUC statistics show diagnostic performance of experiments. ( a ) Shown for biological replicates ( n =3) of control (CTL) and methimazole-treated (MET) from a rat toxicogenomics experiment, ( b ) shown for an RNA-Seq measurement of reference samples (UHRR and HBRR) with library preparation technical replicates ( n =4) from Lab 5 of an interlaboratory study. Annotation tables include AUC statistics for each group of true-positive ERCC controls along with the number of controls that were used in this analysis (‘detected’) and the total number that were included in the ERCC control mixtures (‘spiked’). 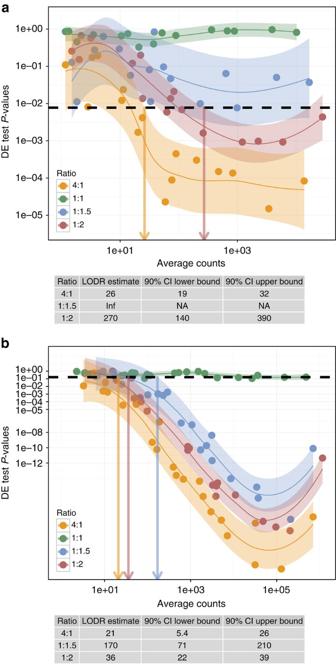Figure 4: Model fits toP-values as a function of average counts are used to estimate LODR. (a) Shown for biological replicates (n=3) of control (CTL) and methimazole-treated (MET) rats with FDR=0.1. (b) Shown for the reference sample RNA-seq experiment technical replicates (n=4) from Lab 5 of an interlaboratory study with FDR=0.01.P-values for these RNA-Seq experiments were from Quasi-Seq differential expression testing. The black dashed line annotates theP-value threshold derived from the FDR chosen for each experiment. Coloured arrows indicate the LODR estimate (average counts) for each fold change that crosses the line indicatingPthreshand the upper boundary of the model 80% confidence interval. LODR results and bootstrap confidence intervals derived from this plot are in the annotation table below the plot. Full size image Figure 4: Model fits to P -values as a function of average counts are used to estimate LODR. ( a ) Shown for biological replicates ( n =3) of control (CTL) and methimazole-treated (MET) rats with FDR=0.1. ( b ) Shown for the reference sample RNA-seq experiment technical replicates ( n =4) from Lab 5 of an interlaboratory study with FDR=0.01. P -values for these RNA-Seq experiments were from Quasi-Seq differential expression testing. The black dashed line annotates the P -value threshold derived from the FDR chosen for each experiment. Coloured arrows indicate the LODR estimate (average counts) for each fold change that crosses the line indicating P thresh and the upper boundary of the model 80% confidence interval. LODR results and bootstrap confidence intervals derived from this plot are in the annotation table below the plot. 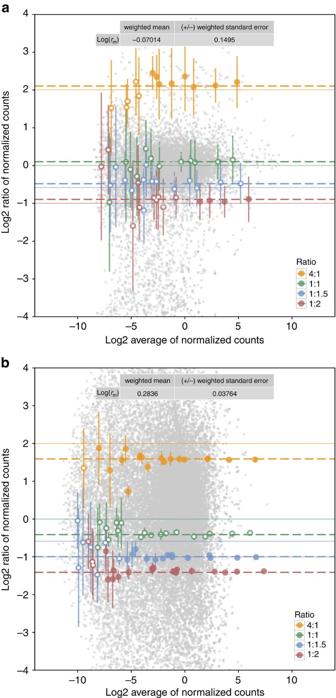Figure 5: MA plots show ratio measurement variability and bias. (a) Shown for biological replicates (n=3) of control (CTL) and methimazole treated (MET) from a rat toxicogenomics experiment. (b) Shown for an RNA-Seq measurement of reference samples (UHRR and HBRR) with library preparation technical replicates (n=4) from Lab 5 of an interlaboratory study. ERCC data points (coloured by ratio) represent the mean ratio measurements per ERCC. Error bars represent the standard deviation of replicate ratios. Filled circles indicate ERCC ratios above the LODR estimate for 4:1, 1:1.5 and 1:2 ratios. Endogenous transcript ratio measurements are shown as grey points. The estimate of mRNA fraction differences between the samples,rm, with weighted standard errors is provided in an inset table and used to adjust the nominal ERCC ratios. The nominal ratios are annotated with solid coloured lines for each ratio subpool and the adjusted ratios are annotated with dashed coloured lines. Full size image Figure 5: MA plots show ratio measurement variability and bias. ( a ) Shown for biological replicates ( n =3) of control (CTL) and methimazole treated (MET) from a rat toxicogenomics experiment. ( b ) Shown for an RNA-Seq measurement of reference samples (UHRR and HBRR) with library preparation technical replicates ( n =4) from Lab 5 of an interlaboratory study. ERCC data points (coloured by ratio) represent the mean ratio measurements per ERCC. Error bars represent the standard deviation of replicate ratios. Filled circles indicate ERCC ratios above the LODR estimate for 4:1, 1:1.5 and 1:2 ratios. Endogenous transcript ratio measurements are shown as grey points. The estimate of mRNA fraction differences between the samples, r m , with weighted standard errors is provided in an inset table and used to adjust the nominal ERCC ratios. The nominal ratios are annotated with solid coloured lines for each ratio subpool and the adjusted ratios are annotated with dashed coloured lines. Full size image Dynamic range of control measurements The 2 20 range of RNA abundance in ERCC Mix 1 and Mix 2 ( Fig. 1b ) is used to assess the dynamic range of an experiment. The rat RNA-Seq experiment has a ~2 15 dynamic range ( Fig. 2a ) and the reference sample RNA-Seq experiment dynamic range spans the 2 20 design dynamic range ( Fig. 2b ). This difference is because of increased sequencing depth in the reference sample experiment. Note that the observed ERCC control signal-abundance relationship ( Fig. 2a,b ) is intended for qualitative assessment of dynamic range. The ERCC controls, as used in these differential gene expression experiments, are not recommended for chemical calibration. The mRNA-enrichment process, in particular poly-A selection, can bias the expected signal-abundance relationship of ERCC controls, which have poly-A tails ranging from ~20 to 26 nt, significantly shorter than endogenous transcript poly-A tails (see Supplementary Figs 21–23 and Supplementary Note 1 ). Diagnostic performance of control ratios When true differences in expression exist between samples in an experiment, those differences should be detected in differential expression tests; where no differences exist, no difference should be detected. The true-positive and true-negative ERCC control ratios can be used in a receiver operator characteristic (ROC) curve analysis of rank-ordered differential expression test P -values ( Fig. 3 ). ROC curves and the corresponding AUC statistics [19] , [20] change based on the discrimination of true-positive values and true-negative values in this rank-ordered list. Perfect diagnostic performance is represented by AUC=1 and a diagnostic failure is indicated by AUC=0.5, meaning that discriminatory power of an experiment is equivalent to a random guess. Within each experiment, there is a predictable increase in diagnostic performance with increasing ERCC ratio differences ( Fig. 3a,b ). This relationship between design ratio and diagnostic performance relies on balanced, matched distributions of positive and negative control abundances. This design requirement is a critical consideration for preparation of any set of external spike-in ratio mixtures for diagnostic performance evaluation. In the rat experiment, all AUC statistics were >0.9, indicating good diagnostic power ( Fig. 3a ). For the reference RNA experiment ( Fig. 3b ), diagnostic performance from ROC curves as AUC statistics is slightly lower. This is explained by the greater sequencing depth in these experiments, resulting in detection of more ERCC controls and a more stringent ROC analysis. This highlights a limitation of ROC curve analysis; it does not directly assess diagnostic performance as a function of abundance. To address this shortcoming, we introduce a new performance measure, LODR estimates. LODR estimates Identifying differentially expressed transcripts is the objective of differential expression experiments; however, how much information (signal) is needed to have confidence that a given fold change in expression of transcripts will be detected? With LODR estimates, empirical ERCC control ratio measurements can inform researchers of diagnostic power at a given fold change relative to transcript abundance for an experiment. An LODR estimate for a particular fold change is the minimum signal, above which differentially expressed transcripts can be detected with a specified degree of confidence. LODR offers a statistically derived, objective alternative to other methods of parsing gene lists. An LODR estimate is obtained for a specified ratio by modelling the relationship between differential expression test P -values and signal. An acceptable false discovery rate (FDR) must be chosen to estimate an LODR. For the selected FDR ( q -value) a threshold P -value can be selected from the population of P -values from the experiment. An LODR estimate for each differential ratio is found based on the intersection of the model confidence interval upper bound (90%) with the P -value threshold. A recommended default for erccdashboard analysis is FDR=0.05; however, this input parameter may be adjusted. For all rat RNA-Seq experiments ( Fig. 4a and Supplementary Figs 1–5 ) FDR=0.1 because in these sequencing experiments the differential expression testing yields P -value distributions that do not contain strong evidence for differences between the samples. A smaller FDR for these experiments would decrease the threshold P -value and increase the LODR estimates. A much lower threshold, FDR=0.01, is used in the reference sample experiments ( Fig. 4b and Supplementary Figs 6–20 ) because large differences in reference sample transcript abundances yield a large number of small P -values. See Methods for more guidance and detail on LODR estimation. In Supplementary Information , we also describe a way to assess validity of the ERCC control data for LODR estimation and an alternative model-based approach for LODR estimation ( Supplementary Figs 24–25 and Supplementary Notes 2–3 ). Detection of differential expression improves with increasing signal for all experiments ( Fig. 4a,b ); this cannot be discerned with ROC analysis. The AUC results for the rat experiment ( Fig. 3a ) had very similar diagnostic performance for all ratios (all ratios have AUC>0.95); however, the LODR estimates for each ratio are significantly different ( Fig. 4a ). This analysis demonstrates that, although AUC statistics can be a good summary of overall diagnostic performance, LODR estimates provide valuable evidence of diagnostic performance with respect to transcript abundance. ERCC results that are above each LODR estimate are annotated with filled points on MA plots [21] ( Fig. 5a,b ); such annotated MA plots can be used to design future experiments to achieve balance between cost and the desired diagnostic power. For example, when signals for genes of interest (GOIs) are observed at or near an LODR estimate, deeper sequencing of the samples should increase signal for the GOIs to be above the LODR estimate. Spike-in control LODR estimates provide an objective expectation for detection of differentially expressed endogenous transcripts but will not substitute for careful experimental design with appropriate biological replication. Bias and variability in control ratio measurements Bias and variability of control ratio measurements are evaluated graphically with MA plots. ERCC control ratio measurements for each of the four ERCC subpools should agree with the nominal ratios (annotated with solid coloured lines in Fig. 5a,b ). The distance between the solid and dashed lines for each ERCC subpool ( Fig. 5a,b ) is the bias in the control ratio measurements. For the rat experiment ( Fig. 5a ), the control ratio measurements show little bias; however, a more significant bias is observed for the control ratio measurements in the reference RNA experiment ( Fig. 5b ). This bias is attributable to the documented difference in mRNA fraction between the two reference samples [22] . Following mRNA enrichment, the relative amount of ERCC mix to endogenous RNA in HBRR is greater than the amount in UHRR; this creates the bias observed in the ERCC control ratio measurements (see example illustration in Supplementary Fig. 26 ). Correcting this bias because of mRNA fraction differences is critical for accurate differential expression testing. A model to describe this bias in control ratios, r m , is: where R S is the nominal ratio of controls in subpool S of a pure ERCC mixture and is the observed ratio of measured ERCC expression values in subpool S in sample 1 and sample 2. In the absence of bias, log( r m )=0. r m should be a property of the samples. An empirical r m value is calculated using the previously reported mRNA fractions of these samples [22] . Deviation from this empirical r m is likely because of bias contributed during sample handling and library preparation procedures (which include mRNA-enrichment procedures). Estimates of log( r m ) derived from erccdashboard analysis for these samples are consistent with this empirical log( r m ) estimate ( Fig. 5b , Supplementary Figs 6–20 ) but with large measurement uncertainties. Recent work has shown that simple normalization approaches can be insufficient for experiments where sample mRNA fractions are significantly different [23] . This work and our analysis here demonstrate the utility of the ERCC controls for the detection of bias in an experiment because of sample mRNA fraction differences. Our analysis presents evidence of bias in ERCC control signals in experiments using poly-A selection for mRNA enrichment ( Supplementary Figs 21–23 and Supplementary Note 1 ). This bias has been reported in earlier work [13] . A protocol-dependent bias (for example, poly-A selection bias) affecting the ERCC control signals prohibits the use of these experimental data for spike-in-based normalization approaches. Deconvolving sample mRNA fraction differences and protocol-dependent bias require experimentally validating the stability of the bias and using this validated protocol. If the protocol-dependent bias is the same (stable) across samples of interest, then normalization using spike-ins should be valid. Any protocol-dependent bias observed with ERCC controls is a red flag that the same bias may affect endogenous transcripts as well. Despite the bias in ERCC control signals arising from inefficiency in their recovery through the mRNA-enrichment process, the ERCC control ratios are stable and useful for measurement assurance of endogenous transcript ratio measurements. We observed that samples treated in the same library preparation batch experienced the same protocol-dependent bias. All transcript ratios were calculated between samples within a single library preparation batch and the ERCC ratio results are shown to be precise and stable across a broad dynamic range and multiple ratios ( Fig. 5a,b and Supplementary Figs 1–20d ). ERCC ratio measurements in the reference sample experiments have smaller variability compared with the rat experiment measurements. This difference in ratio variability can be attributed to both lower sequencing depth in the rat experiment as well as variability in spiking these biological samples (reference samples were spiked once in bulk and then aliquoted). Application of the erccdashboard: interlaboratory analysis Interlaboratory reproducibility of RNA-Seq experiments is evaluated by comparing erccdashboard performance measures using the spiked reference RNA samples. Three different measurement processes (sample preparation and sequencing platform) were used at different laboratories: Illumina SEQC sequencing sites (ILM SEQC Lab 1–6), Life Technologies SEQC sequencing sites (LIF SEQC Lab 7–9) and Illumina ABRF sequencing sites (ILM ABRF Lab 10–12). At the ILM ABRF sites, ribosomal RNA depletion was used for mRNA enrichment. At ILM SEQC and LIF SEQC sites, reference sample total RNA went through two rounds of poly-A selection but a different type of kit and experimental protocol was used for each platform. Poly-A selection was carried out independently for each library replicate at ILM SEQC sites, and at LIF SEQC sites poly-A selection was carried out for each sample type. While reproducibility can be evaluated with these experiments, note that strong conclusions regarding performance of particular laboratories, sample preparation protocols or sequencing platforms (these factors are confounded) would require a more systematic study design repeated over time. LODR estimates complement AUC statistics for each interlaboratory site ( Fig. 6a,b ), supporting the use of the more informative LODR as a new performance metric. For the ILM SEQC experiments (Lab 1–6), although the AUC statistics for all ratios at Lab 2 indicate slightly decreased diagnostic performance, the LODR estimates showed similar performance across all six sites. LODR estimates from the ILM ABRF experiments were consistent with ILM SEQC experiments despite lower AUC statistics for the ILM ABRF experiments (Lab 10–12). For the LIF SEQC experiments (Lab 7–9), both the AUC statistics and LODR estimates indicated reduced diagnostic performance at Lab 7. For 1:1.5 ratio measurements in this experiment, diagnostic performance is very poor, AUC <0.7, and an LODR estimate could not be obtained for the specified FDR. 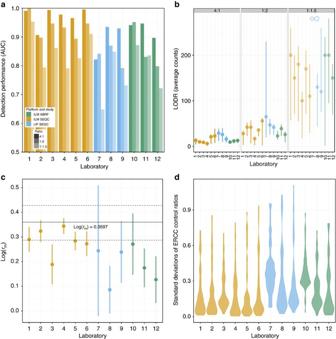Figure 6: Interlaboratory comparison of erccdashboard performance measures for reference sample experiments. (a) AUC statistics are shown for the ERCC controls at the three differential ratios. (b) LODR count estimates (on a log scale) for the ERCC controls at the three differential ratios. Error bars represent LODR bootstrap method 90% confidence intervals. (c) Weighted mean estimates of mRNA fraction differences for the sample set with error bars representing weighted standard errors. The solid black line represents the measurement ofrmfrom previous work22and dashed black lines show the confidence interval from the standard deviation of this estimate. (d) Violin plots show distributions of ERCC control ratio standard deviations at each laboratory. The legend is common to all figures, colour indicates measurement process and transparency of each colour is used to indicate results for different ratios. Figure 6: Interlaboratory comparison of erccdashboard performance measures for reference sample experiments. ( a ) AUC statistics are shown for the ERCC controls at the three differential ratios. ( b ) LODR count estimates (on a log scale) for the ERCC controls at the three differential ratios. Error bars represent LODR bootstrap method 90% confidence intervals. ( c ) Weighted mean estimates of mRNA fraction differences for the sample set with error bars representing weighted standard errors. The solid black line represents the measurement of r m from previous work [22] and dashed black lines show the confidence interval from the standard deviation of this estimate. ( d ) Violin plots show distributions of ERCC control ratio standard deviations at each laboratory. The legend is common to all figures, colour indicates measurement process and transparency of each colour is used to indicate results for different ratios. Full size image Weighted mean estimates of the mRNA fraction difference between the UHRR and HBRR samples for the ILM SEQC experiments generally show agreement with the previously reported r m measurement ( Fig. 6c ) with the exception of Lab 3. This lab also had an increased standard error for r m compared with the other ILM SEQC labs. This difference is echoed in other upstream QC analysis of the ILM SEQC data that showed decreased sequencing read quality at Lab 3 (refs 17 , 24 ). Large standard errors for r m were obtained for the laboratories in both the ILM ABRF and LIF SEQC experiments. This increased variability in the r m estimates is echoed in violin plots of ratio standard deviations at each site ( Fig. 6d ). In the ILM ABRF experiments, Lab 10 had particularly high ratio measurement variability, suggesting the presence of a batch effect at this site (See also Supplementary Fig. 24 and Note 2 ). At Lab 7 in the LIF SEQC experiments, the r m estimate standard errors and overall ratio measurement variability were very high ( Fig. 6c,d ), and this site also showed poor diagnostic performance ( Fig. 6a,b ). QC metrics show consistency for within-platform differences Analysis of the ERCC control ratio ‘truth set’ provides evidence of the poor ratio measurement performance in the Lab 7 differential expression experiment; however, technology-specific QC measures are needed to link observations of poor ratio measurement performance to upstream causes such as sample preparation issues. QC assessment of the mapped read data for the three Life Technologies sites was used to identify possible reasons for performance differences in these experiments. Lab 7 performance is not an artifact of read mapping and quantification; similar results were obtained for LIF SEQC data using both the Life Technologies LifeScope analysis pipeline ( Supplementary Figs 12–14 ) and the Subread [25] and featureCounts [26] analysis pipeline ( Supplementary Figs 27–29 ). Mapped read QC metrics from RNASeQC [9] for a small subset of UHRR data from Lab 7–9 mapped with LifeScope show possible reasons for performance differences. Lab 7 had an increased percentage of duplicated reads in the libraries they prepared; a fifth library prepared at an independent site (and then shared among the three laboratories for sequencing) showed a lower duplication rate ( Supplementary Fig. 30 ). These results suggest that libraries prepared at Lab 7 had low complexity. Evidence for 3′ coverage bias is observed across all libraries for the middle 1,000 expressed transcripts ( Supplementary Fig. 31 ). For the top 1,000 expressed transcripts, the four libraries prepared at Lab 7 showed increased 3′ coverage bias relative to the four libraries prepared at Lab 8 and 9 ( Supplementary Fig. 32 ). There were no significant differences in ribosomal RNA mapping fractions for libraries 1–4 at the three laboratories ( Supplementary Fig. 33 ). The erccdashboard R package is a method validation tool for standard analysis of differential gene expression experiments. The key technical performance parameters from ERCC control ratio mixtures are evaluated with four main analysis figures produced by the software. Examples of these four figures are shown for two different experiment types in Figs 2 , 3 , 4 , 5 . These technology-agnostic performance measures include dynamic range, diagnostic performance, LODR estimates and expression ratio bias and technical variability. A dynamic range of 2 16 is desirable as a general rule of thumb for a typical RNA-Seq gene expression experiment. The best observable dynamic range with the ERCC control ratio mixtures used in this study is 2 20 . Diagnostic performance of an experiment can be assessed with ROC curve analysis; however, care should be taken in comparison of AUC statistics across experiments without consideration of the number of controls detected in each experiment. An experiment with 4:1 AUC of 0.85 where 16 controls were detected out of 23 spiked controls may not necessarily have better performance than an experiment where 23 controls were detected and the 4:1 AUC is 0.8. This and other issues noted for ROC curve analysis [20] underscore the benefit of using the new LODR performance metric that summarizes diagnostic performance with respect to abundance in any experiment and can be informative for experimental design. If signals from the GOIs in a study are above the LODR then that indicates the sequencing depth is sufficient. When this is not the case, deeper sequencing of the samples should increase signal for the GOIs to be above the LODR estimate. Statistically significant ratio measurement bias indicates an experimental artifact (for example, protocol-dependent bias) or an mRNA fraction difference between samples. The source of bias should be identified and addressed with validated methods. Most reference RNA experiments had a ratio measurement bias that could be explained by the known mRNA fraction difference for the reference RNA samples; however, several experiments showed a significant difference, and some had very large standard errors. For these experiments, there may be other batch effects that shifted the ratio measurement bias or contributed to the large standard errors. These differences between experiments highlight the utility of ERCC ratio measurements as a truth set to benchmark the accuracy of endogenous transcript ratio measurements. In other words, ERCC ratio bias in an experiment suggests that endogenous transcript ratios may be biased in that experiment as well. Our analysis tool based on the ERCC controls provides researchers with the ability to use empirical evidence to assess bias in an experiment that may affect both controls and endogenous transcripts. Without the use of appropriate controls and related analysis methods, the presence of such bias might remain undetected. Method validation can be accomplished with these ERCC ratio performance measures for any gene expression measurement technology, including both RNA-Seq and microarrays, which can give comparable differential expression results with appropriate experimental design and analysis. Reproducible research calls for standard approaches to assess, report and compare the technical performance of genome-scale differential expression experiments. As measurement technology costs decrease, differential expression measurements are increasing in scope and complexity, including experimental designs with large sample cohorts, measured over time, at multiple laboratories. Even a single canonical differential expression experiment can involve the effort of multiple investigators, from the experimentalist generating the samples and eventually reporting the conclusions to the many scientists performing sample preparation, sequencing, bioinformatics and statistical analysis. These erccdashboard performance measures provide a standard method to enable the scientific community conducting differential expression experiments to critically assess the performance of single experiments, performance of a given laboratory over time or performance among laboratories. Standard method validation of experiments with erccdashboard analysis will provide scientists with confidence in the technical performance of their experiments at any scale. Reference RNA sample preparation and RNA-Seq The two ERCC spike-in RNA transcript mixtures (Ambion, Life Technologies) were produced from plasmid DNA templates (NIST Standard Reference Material 2374). The reference RNA samples, Universal Human Reference RNA [16] (Agilent Technologies) and Human Brain Reference RNA (Ambion, Life Technologies) were spiked with the two ERCC spike-in RNA transcript mixtures (Ambion, Life Technologies) by FDA National Center for Toxicological Research and distributed to SEQC site laboratories for sequencing on Illumina, Life Technologies, and Roche platforms as described in the main SEQC project manuscript [17] and these samples were also used in the ABRF interlaboratory study [18] . In brief, 50 μl of ERCC Mix 1 was spiked into 2500 μl UHRR (Universal Human Reference RNA) total RNA and 50 μl ERCC Mix 2 was spiked into 2,500 μl HBRR (Human Brain Reference RNA) total RNA. Single aliquots (10 μl each) of these two samples were sent to each participating laboratory to produce replicate library preparations of samples. For the SEQC study, there were separate library preparation protocols for the Illumina and Life Technologies platforms including different poly-A selection protocols for mRNA enrichment. Replicate library preparations ( n =4) were prepared at every laboratory and then at each laboratory all library preparations were barcoded, pooled and sequenced with 2 × 100 paired-end sequencing chemistry for Illumina and 50 × 35 paired-end sequencing chemistry for Life Technologies using the full fluidic capacity of an instrument (all lanes and flow cells). Experiments for SEQC interlaboratory analysis from six Illumina sites and three Life Technologies sites were compared in this analysis. In addition to the SEQC data, we also evaluated three Illumina sequencing experiments from the ABRF study that used ribo-depletion for mRNA enrichment instead of poly-A selection. In these experiments, replicate library preparations ( n =3) were sequenced at each laboratory with 2 × 50 paired-end sequencing chemistry. For the Illumina SEQC reference RNA libraries, the mean number of reads per library was 260,098,869 reads, for the Life Technologies SEQC reference RNA libraries the mean number of reads per library was 109,307,746 reads and for the ABRF Illumina reference RNA libraries the mean number of reads per library was 257,451,483 reads. Rat toxicogenomics sample preparation and RNA-Seq Library preparation for rat toxicogenomics study samples was performed at a single laboratory with sequencing runs on Illumina HiScanSQ and HiSeq 2000 instruments as described in the companion rat toxicogenomics manuscript [14] . A subset of data, measured with the HiScanSQ, was analysed here. Rats in the MET, 3ME and NAP sample sets were treated orally with met himazole, 3-me thylcholanthrene, and beta nap thoflavone, and compared with the same set of control rats. Rats in the THI and NIT sample sets were treated by injection with thi oacetamide and N- nit rosodimethylamine. RNA samples from treated rat replicates were spiked with ERCC Mix 1 (per treatment type n =3). We retained the match control (CTL) samples that were spiked with ERCC Mix 2; for the MET, 3ME and NAP experiments, there were n =3 CTL samples and for the THI and NIT experiments the three CTL samples with the highest RIN numbers were used from a set of five CTL samples. For the five rat toxicogenomics experiments (21 samples), the mean number of total reads per library was 40,281,946 reads. Bioinformatic analysis of RNA-Seq experiments Rat toxicogenomics sample data were mapped at the National Center for Toxicological Research against rat and ERCC reference sequences using Tophat [27] . Sequence reads from the SEQC interlaboratory study were aligned to human (hg19) and ERCC reference sequences. SEQC study Illumina platform data were mapped with Burrows-Wheeler Aligner (BWA) [28] and gene level counts corresponding to human and ERCC nucleic acid features were quantified using reference annotations for the ERCC controls and hg19 (NCBI RefSeq, Release 52). SEQC study Life Technologies platform data were mapped with LifeScope (Life Technologies, Foster City, CA, USA) and reference annotations from UCSC and NIST. Life Technologies platform data were also mapped with the Subread aligner [25] and summarized using the featureCounts programme [26] . ABRF Illumina data used in this analysis were mapped with the STAR aligner using the hg19 genome assembly, and the Gencode v12 annotation was used for read counting with the Rmake pipeline ( http://physiology.med.cornell.edu/faculty/mason/lab/r-make/ ). Count data from these experiments were used in the erccdashboard analysis. The default normalization for all RNA-Seq experiment sample replicates was 75th percentile normalization of count data. Reference RNA microarray analysis In the SEQC study, there were three microarray experiments. Two experiments used Illumina Bead Arrays (Lab 13 and 14). For Lab 13 and 14, triplicate arrays were prepared for each reference RNA sample. Microarray signal intensity data were not background-corrected or normalized using the Illumina software. The unnormalized data were processed to keep only the results in all sample replicates ( n =6) that had probe detection P -values that were ⩽ 0.05. In erccdashboard analysis, the replicates in these array experiments were normalized using the 75th percentile intensity for each replicate array. At Lab 15, custom Agilent 1 M microarrays ( n =4 per sample) with a variance stabilizing normalization [29] were used in erccdashboard analysis. For the Agilent arrays, probe sequence-specific signals were modelled using established methods, saturation effects detrended and outlier probes downweighted [30] , [31] , [32] . Gene expression data analysis with the erccdashboard The erccdashboard software package was developed in the R statistical computing language [33] and the package is freely available from GitHub ( https://github.com/usnistgov/erccdashboard ) and Bioconductor [34] . The erccdashboard package documentation includes a user guide to describe how to use the software for analysis of gene expression data. A negative binomial generalized linear model was fit to counts for individual ERCC controls from each replicate of the treatment and control samples to estimate the bias in the empirical ERCC ratios ( r m ). These individual ERCC r m estimates and standard errors were used to produce an overall weighted mean r m estimate with a weighted standard error estimate. The r m estimate must be applied as a correction factor to ERCC data before further analysis. For RNA-Seq experiments, differential expression testing of ERCCs and endogenous genes was performed with QuasiSeq [35] , using a negative binomial dispersion trend estimated from edgeR [36] , [37] , to generate P -values for all endogenous and ERCC features. For microarray experiments, limma [38] was used for differential expression testing. ROC curves and AUC statistics were produced using the ROCR package [39] . To construct the ROC curves, the 1:1 subpool P -values were the true-negative group for each differential ratio ROC curve. Estimation of LODR requires the following parameters: fold change, fold ; probability, prob ; and P -value threshold, p thresh . An LODR estimate is defined as the minimum count above which a transcript with an absolute log fold change, |log(fold)|, has at least a prob *100% chance of obtaining a q -value of FDR or less. The choice of p thresh is based on specification of an acceptable FDR, typically this may be FDR =0.05, but for samples with higher or lower populations of differentially expressed genes one can be more or less conservative in this choice. In our analysis, FDR=0.1 was used to compare all rat data sets and FDR=0.01 was used for all human reference RNA data sets. For each P -value obtained from differential expression testing of the population of transcripts a q -value (estimated FDR) is computed. The maximum P -value that has a corresponding q -value less than or equal to FDR is defined as p thresh . LODR estimates for each of the differential ERCC ratios were made using locfit [40] regression trends (including a pointwise 80% prediction interval) of the relationship between abundance (log10(average count)) and strength of differential expression (log10( P -value)). For a given fold (ratio), the LODR is the average count where the upper bound of ratio prediction interval intersects with a chosen p thresh . This method of estimating LODR is annotated with coloured arrows in Fig. 4 . For each LODR estimate, 90% confidence intervals were obtained via bootstrapping (residuals from the corresponding locfit curve were repeatedly resampled to estimate LODR). For evaluating ratio measurement variability for the pair of samples in an experiment, ratios of ERCC control signals for the samples were examined with respect to the average of the sample ERCC control signals. MA plots of these data were annotated to indicate ERCC ratio measurements above and below the LODR estimates for each ratio. Violin plots of the density distribution of ERCC control ratio s.d.’s (with the upper 10th percentile trimmed) are used to evaluate ratio measurement variability for multiple experiments. All diagnostic plots provided by the erccdashboard tool were generated based on tools available in the ggplot2 (ref. 41 ) and gridExtra [42] R packages. Mapped read QC analysis Mapped read QC metrics were produced for Life Technologies data from Lab 7 to 9. The percentage of rRNA mapped in all UHRR Libraries (1–5) technical replicates (all lanes and flow cells) at Lab 7-9 were extracted from LifeScope mapping filter reports that result from sample alignment to a reference file of filter reference sequences. A subset of UHRR Library 1-5 bam files that were each downsampled to approximately one million read pairs using the downSampleSam function in Picard [43] were analysed using the RNASeQC analysis tool [9] to assess duplicate read rates and coverage bias across transcripts. Data access Sequence data used in this analysis are from the SEQC manuscripts [14] , [17] and the ABRF study manuscript [18] . The full SEQC project data set has been deposited in GEO and is accessible by the code GSE47792 and the full ABRF study data set is accessible by the code GSE46876. Expression measure tables derived from the RNA-Seq and microarray data are available ( Supplementary Data 1 ) so that the analysis presented here may be reproduced in R with the erccdashboard package. How to cite this article: Munro, S. A. et al . Assessing technical performance in differential gene expression experiments with external spike-in RNA control ratio mixtures. Nat. Commun. 5:5125 doi: 10.1038/ncomms6125 (2014).